Carbon nanotubes asin vivobacterial probes With the rise in antibiotic-resistant infections, non-invasive sensing of infectious diseases is increasingly important. Optical imaging, although safer and simpler, is less developed than other modalities such as radioimaging, due to low availability of target-specific molecular probes. Here we report carbon nanotubes (SWNTs) as bacterial probes for fluorescence imaging of pathogenic infections. We demonstrate that SWNTs functionalized using M13 bacteriophage (M13-SWNT) can distinguish between F′ -positive and F′ -negative bacterial strains. Moreover, through one-step modification, we attach an anti-bacterial antibody on M13-SWNT, making it easily tunable for sensing specific F′ -negative bacteria. We illustrate detection of Staphylococcus aureus intramuscular infections, with ~3.4 × enhancement in fluorescence intensity over background. SWNT imaging presents lower signal spread ~0.08 × and higher signal amplification ~1.4 × , compared with conventional dyes. We show the probe offers greater ~5.7 × enhancement in imaging of S. aureus infective endocarditis. These biologically functionalized, aqueous-dispersed, actively targeted, modularly tunable SWNT probes offer new avenues for exploration of deeply buried infections. Bacterial infections are one of the leading causes of mortality and morbidity globally [1] . According to US data, bacterial infections result in thousands of deaths due to sepsis and limb amputations [2] , [3] , with an estimated economic impact of ~$5–$24 billion [4] annually. Despite the availability of antibiotics, a major challenge in the effective treatment of bacterial infections is the inability to detect them in vivo with high sensitivity and specificity. Further, the large increase in the development of antibiotic-resistant bacterial strains necessitates a search for more sophisticated imaging modalities for early sensing of infections, with better chances of therapy [1] . Currently, targeting via ex vivo radiolabelled autologous leukocytes, developed in the 1970s to 1980s, is still considered the ‘gold standard’ nuclear medicine technique for imaging of infectious diseases [5] , [6] . However, this approach exposes the patient to radiation, is laborious to design and implement, requires specialized equipment including sources/detectors and operator training. In contrast, optical imaging offers the advantages of being a relatively safe method, using non-ionizing light sources, simple-to-design and operate equipment; making it more suitable for deployment in rural areas and mobile clinics even in less affluent communities. Although genetic reporters, including light-emitting luciferase enzymes or fluorescent proteins such as green fluorescent protein [7] , have been used for optical imaging of infections in vivo , they are not endogenously expressed by most naturally occurring pathogens. Several groups have explored exogenous agents such as antibodies [8] , sugars, lectins, antibiotic drugs, antimicrobial peptides [9] , [10] , cationic charged cell membrane-penetrating peptides [11] , [12] and specially designed molecules [13] , [14] , [15] for targeting bacteria. However, for many of these targeting agents, the success is limited by their specificity, due to the possibility of the affinity ligand targeting the necrotic tissue produced around the site of infection [13] , [14] . Recent work on fluorescently labelled sugars internalized through bacteria-specific transport pathways [16] has shown good promise for specific targeting of bacterial pathogens. Among these methods, antibody-based probes are attractive due to their modularity, specificity and high affinity to surface antigens present on both Gram-positive and Gram-negative bacteria, and offer the potential of improved targeting. In recent years, optical imaging using fluorescence emission in the second-window near-infrared (NIR-II: 900–1,400 nm) regime has emerged as a promising domain for in vivo imaging, fueled by the development of better molecular probes, effective targeting agents [17] and custom-built imagers [17] , [18] , [19] . NIR-II light can penetrate biological tissue more efficiently with less tissue scattering than visible and first-window near-infrared (NIR-I: 650–900 nm) light [20] , [21] . Reports suggest maximum achievable penetration depth in living tissue to be in the 1,000–1,400 nm wavelength range [22] , [23] , [24] , with a potential 100-fold improvement in signal-to-noise than NIR-I. Single-walled carbon nanotubes (SWNTs) are an attractive candidate as fluorophores for NIR-II imaging, due to their photoluminescence in the 900–1,400 nm range, large Stokes’ shift, low-autofluorescence background, relative insensitivity to photobleaching compared with organic dyes, ability to be functionalized with targeting/drug delivery agents and high optical absorbance in NIR-I offering the additional possibility of photothermal therapy. Although SWNTs have been used previously for fluorescence imaging of cells [17] , tumours [19] , for dynamic contrast imaging [18] , or vascular imaging [25] and photothermal therapy [26] , the application of SWNT probes for actively targeted fluorescence imaging of bacterial infections in vivo has not yet been realized, to the best of our knowledge. It is critical to form a stable aqueous dispersion of hydrophobic SWNTs for bioimaging applications, to functionalize and render them biocompatible, prevent agglomeration and retain their photoluminescence properties and add moieties for effective targeting. Our group has developed M13 bacteriophage as a biological scaffold capable of simultaneously functionalizing and dispersing SWNTs in aqueous media [27] . M13 is a filamentous, non-lytic bacteriophage with dimensions ~880 nm in length and ~6 nm in diameter. The five surface capsid proteins (p3, p5, p7, p8 and p9) of M13 can be genetically engineered to display peptides with multiple functionality such as targeting motifs against tumour cells [28] , [29] and load drug molecules or fluorescent probes [30] . Specifically, we have shown the major coat protein p8 can functionalize SWNTs through a multivalent, high-copy, longitudinal π – π interaction [27] . This M13-SWNT conjugate maintains sufficient fluorescence activity and can be deployed for high-quality NIR-II imaging of living subjects. Further, M13 is an excellent candidate for detecting bacterial infections due to its natural binding affinity to bacteria, which express F′ -pili, and its ability to be easily tuned for specific targeting of numerous other F′ -negative bacterial strains. In this work, we present biologically functionalized, aqueous-dispersed, actively targeted SWNTs as modularly tunable, highly specific probes for non-invasively detecting, imaging and monitoring bacterial pathogens in living hosts. We have engineered M13 as a multifunctional platform capable of dispersing SWNTs in a stable aqueous suspension, and tailored the minor coat protein p3 in a one-step tuning process for site-specific attachment of antibodies able to target multiple strains of bacteria. This antibody-labelled SWNT probe shows high specificity of targeting models of infection in live animals, which is validated through ex vivo tissue analyses and histology. In addition, using phantom models of tissue, we show that our probes based on SWNT NIR-II fluorescence offer significantly higher signal amplification, and much lower areal spread at greater depths in tissue, compared with common NIR-I dyes. Further, using a mouse model of bacterial endocarditis we demonstrate that our SWNT probes offer high-contrast, highly specific detection of deeply buried infections. This study opens up exciting new possibilities for deep-tissue optical imaging using SWNT probes, which may be challenging to achieve using conventional dye-based fluorophores. 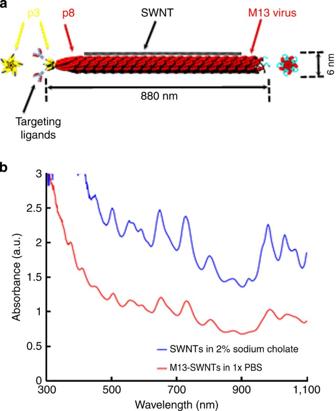Figure 1: Schematic of the SWNT probe and its absorbance spectrum. (a) Structure of the SWNT probe. M13 is a filamentous, cylindrical bacteriophage, rendered in red, with typical dimensions ~880 nm in length and ~6 nm in diameter. Of interest is the major coat protein, p8, which can be used to longitudinally functionalize SWNTs, shown in black, and the minor coat protein, p3, which can be used to bind targeting ligands such as antibodies. (b) Absorbance spectra of aqueous-dispersed SWNTs; using 2 wt% sodium cholate, an organic surfactant (blue curve), and after surfactant exchange to form the M13-SWNT complex (red curve). The characteristic peaks are maintained, although there is slight red shift in the M13-SWNT spectrum. Aqueous functionalized SWNT probes Figure 1a shows the typical structure of the M13 virus used to functionalize SWNTs (M13-SWNT complex). Absorbance spectrum was measured to quantify the effective concentration of SWNTs, illustrated in Fig. 1b . Initially, the SWNTs were aqueous-dispersed using 2 wt% sodium cholate (SC-SWNT), an organic surfactant (blue curve), giving a value of [SWNTs]=58.46 μg ml −1 . After doing the surfactant-exchange process [27] in which the M13-SWNT complex forms, the absorbance spectrum of M13-SWNT (red curve) gives an effective concentration of [SWNTs]=28.64 μg ml −1 . It is observed that after complexation, M13-SWNT shows the same qualitative peak characteristics as the starting SC-SWNTs. There is slight red shifting of the M13-SWNT peaks compared with SC-SWNTs, which may be attributed [19] to the change in the dielectric environment surrounding the SWNTs on conjugation with M13, or due to potentially small amount of bundling of the SWNTs during the complexation process. For additional characterization, including high-resolution transmission electron microscopy and photoluminescence emission spectra images, see Supplementary Fig. 1 and Supplementary Note 1 of Supplementary Information . Figure 1: Schematic of the SWNT probe and its absorbance spectrum. ( a ) Structure of the SWNT probe. M13 is a filamentous, cylindrical bacteriophage, rendered in red, with typical dimensions ~880 nm in length and ~6 nm in diameter. Of interest is the major coat protein, p8, which can be used to longitudinally functionalize SWNTs, shown in black, and the minor coat protein, p3, which can be used to bind targeting ligands such as antibodies. ( b ) Absorbance spectra of aqueous-dispersed SWNTs; using 2 wt% sodium cholate, an organic surfactant (blue curve), and after surfactant exchange to form the M13-SWNT complex (red curve). The characteristic peaks are maintained, although there is slight red shift in the M13-SWNT spectrum. Full size image We performed in vitro plate assays to determine the binding capability of the SWNT probe, to Escherichia coli and S. aureus cell lines (see Supplementary Fig. 2 and Supplementary Note 2 ). The targeted SWNT probe shows up to ~4.2 × enhancement in the fluorescence intensity over the non-targeted case and is sensitive enough to be significantly detected at up to 16 × dilution factor of the stock concentration. This ability to form a strong, multivalent binding to fluorescent SWNTs without complete quenching through biological functionalization on a single vector (M13) while retaining additional handles for achieving targeting and signal amplification at the site of bacterial infection is one of the key advantages of our M13-SWNT system. Whole animal imaging using tunable SWNT probes M13 virus has a natural binding affinity towards certain strains of E. coli , which express F′ -pili appendages. To evaluate the targeting capability of the M13-SWNT complex, we first performed a study of an infection model using E. coli . Two groups of mice ( N =5 each) were infected intramuscularly on their right flank, with one group receiving the F′ -negative DH5-α strain and the other group receiving the F′ -positive JM109 strain. As a control, we also injected PBS intramuscularly in the left flank of all mice. After incubating the bacteria, we injected the M13-SWNT probe intravenously. The time of injection of the probe was taken as t =0. Based on a suitable uptake period typical to most studies [13] , [14] , [16] of imaging of infections, we imaged the mice at t =24 h post injection (p.i.) using a custom-built NIR-II fluorescence imager [19] (see Supplementary Fig. 3a and Supplementary Note 3 for details). All NIR-II fluorescence images have been corrected to account for tissue autofluorescence background, averaged from a control, uninfected, undosed mouse ( Supplementary Fig. 3c,f and Supplementary Note 3 ). 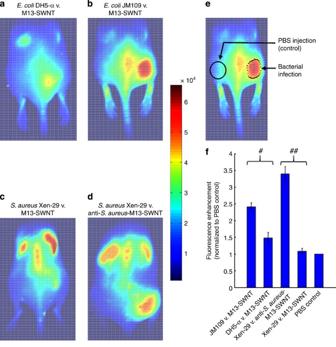Figure 2: Specificity of the SWNT probe. One representative mouse (out ofN=5) from each group is shown here. Mice infected withE. colistrains (a)F’-negative DH5-α, and (b)F’-positive JM109. Both mice received the M13-SWNT probe for imaging. In the lower panel, both mice were infected withS. aureusstrain Xen-29. Mouse (c) received M13-SWNT, while mouse (d) received the targeted anti-S. aureus-M13-SWNT probe injection. (e) Representative image of RoI analyses. For the right flank (site of infection), a thresholding function was used, with a cutoff 35% of peak intensity. For the left flank (control PBS injection), an equi-areal circular RoI was used. (f) Intensity enhancement of the fluorescence signal over the RoI, normalized to baseline intensity (PBS control, left flank). Data plotted as mean±s.d. forN=5 measurements. #,##P<0.01; statistically significant using Student’st-test. Figure 2a,b show representative images of the two groups of mice. Region of interest (RoI) analyses were performed to determine the average enhancement in fluorescence signal intensity over the background (control PBS injection) case, with an example shown in Fig. 2e . The results are plotted in Fig. 2f , normalized with respect to the control PBS injections. We see a signal enhancement ~2.4 × in the targeted JM109 case, which corresponds to a ~1.6 × increase over the non-targeted DH5-α case. These observations are statistically significant and demonstrate good targeting specificity of M13 to F′ -positive strains. Figure 2: Specificity of the SWNT probe. One representative mouse (out of N =5) from each group is shown here. Mice infected with E. coli strains ( a ) F’ -negative DH5-α, and ( b ) F’ -positive JM109. Both mice received the M13-SWNT probe for imaging. In the lower panel, both mice were infected with S. aureus strain Xen-29. Mouse ( c ) received M13-SWNT, while mouse ( d ) received the targeted anti- S. aureus -M13-SWNT probe injection. ( e ) Representative image of RoI analyses. For the right flank (site of infection), a thresholding function was used, with a cutoff 35% of peak intensity. For the left flank (control PBS injection), an equi-areal circular RoI was used. ( f ) Intensity enhancement of the fluorescence signal over the RoI, normalized to baseline intensity (PBS control, left flank). Data plotted as mean±s.d. for N =5 measurements. #, ##P <0.01; statistically significant using Student’s t -test. Full size image However, many strains of bacteria commonly found in the clinical setting lack F′ -pili. Therefore, to make the SWNT probe more widely suitable for detecting other strains, we devised a one-step tuning procedure (see Methods). Employing a genetically engineered form of M13 that expresses biotin-acceptor peptide [19] on the p3 coat protein, we attached a specific anti-bacterial antibody on the p3 through a streptavidin-biotin reaction. This one-step modular process opens up tremendous opportunities for using SWNTs as probes to selectively target and image numerous strains of bacteria, against which antibodies are available. Here we study this using an infection model of S. Aureus , which is F′ -negative, but a dreaded clinical pathogen. Two groups of mice ( N =5 each) received intramuscular infections of S. aureus strain Xen-29 in their right flank and control PBS injections in the left flank. After incubating the bacteria, the first group of mice received an intravenous dose of the nonspecific M13-SWNT probe. In contrast, the second group received the targeted, anti- S. aureus antibody-labelled probe, hereafter referred to as anti- S. aureus -M13-SWNT. For active targeting, we expect the rate of uptake at the site of infection and clearance from the general circulation to be faster, based on reports of M13-based probes used in tumour imaging applications [19] , [29] . We therefore imaged these groups of mice at t =8 h p.i. Figure 2c,d show one representative mouse from each of these cohorts. From the RoI analysis in Fig. 2f , we observe a much greater ~3.4 × enhancement in the fluorescence signal for the targeted case (Xen-29 v. anti- S. aureus -M13-SWNT), which corresponds to a ~3.1 × increase in intensity over the nonspecific case (Xen-29 v. M13-SWNT). We also show detection at lower levels of infection (see Supplementary Fig. 4 and Supplementary Note 4 ). These results establish the specificity of the SWNT probe, with improved signal-to-background contrast for imaging in live subjects. It is also worth noting here that our SWNT probe dosage, ~29 μg ml −1 , is up to an order of magnitude lower than the ~100–500 μg ml −1 bolus of SWNT-based probes reported to be used [17] , [18] , [25] , [26] , [31] in other in vivo applications. Ex vivo analysis using histology and microscopy To reduce the effects of tissue autofluorescence background for corroborative ex vivo analyses and eliminate false-positive results, we euthanized the mice after completing the imaging sequence. Tissue samples were excised and imaged, both from the right thigh muscle (site of infection) and left thigh (control PBS injection), shown in Fig. 3 . As examples, Mouse 1 ( Fig. 3a ) received anti- S. aureus -M13-SWNT, while Mouse 4 ( Fig. 3b ) received the non-targeted M13-SWNT probe, with L and R referring to the left and right thigh, respectively. 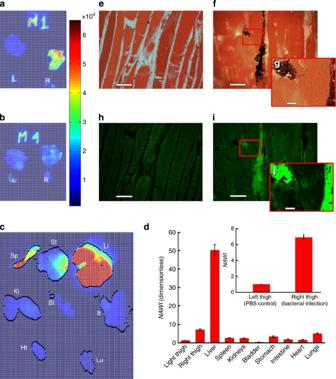Figure 3:Ex vivoanalyses of targeting of the SWNT probe. Mice were euthanized att=24 h post injection (p.i.) after the imaging sequence was completed. (a,b) Representative muscle tissue, denoting the right flank (R, site of infection) and the left flank (L, PBS control). (a) Mouse 1 received the targeted anti-S. aureus-M13-SWNT probe, while (b) Mouse 4 was injected non-targeted M13-SWNT probe. (c) Excised organs;Sp: Spleen,St: Stomach,Li: Liver,Ki: Kidneys,Bl: Bladder,It: Intestine,Ht: Heart,Lu: Lungs. (d) NAWI plot showing relative distribution of the probe, as mean ±s.e.m. forN=5 observations. See Methods for definition of NAWI. Inset is magnified for the thigh muscle tissues, showing a ~6.9 × increase in the probe accumulation at the site of infection. (e–j) Microscopy analysis of excised muscle tissue. (e–g) Bright-field images, with Gram staining. (h–j) Fluorescence images, using a green dye labelled on the M13. (e,h) The left muscle (control PBS injection) shows no evidence of Gram-positiveS. aureusbacteria and negligible green fluorescence. (f,i) The right muscle (site of infection) shows the presence of clumps of violet-stained cocci ofS. aureus. There is marked enhancement in the fluorescence intensity in the regions of large bacterial infection. Insets to parts offandi, indicated by the red boxes, are shown ingandjrespectively, at × 100 magnification. Ing, individual cocci, ~0.5–0.8 μm in diameter are resolved. Inj, the more heavily infected area shows brighter fluorescence compared with the less infected region. SeeSupplementary Fig. 7andSupplementary Note 7ofSupplementary Informationfor additional analysis. Scale bar, 67.5 μm (e,f,h,i) and 13.7 μm (g,j). Figure 3: Ex vivo analyses of targeting of the SWNT probe. Mice were euthanized at t =24 h post injection (p.i.) after the imaging sequence was completed. ( a , b ) Representative muscle tissue, denoting the right flank ( R , site of infection) and the left flank ( L , PBS control). ( a ) Mouse 1 received the targeted anti- S. aureus -M13-SWNT probe, while ( b ) Mouse 4 was injected non-targeted M13-SWNT probe. ( c ) Excised organs; Sp : Spleen, St : Stomach, Li : Liver, Ki : Kidneys, Bl : Bladder, It : Intestine, Ht : Heart, Lu : Lungs. ( d ) NAWI plot showing relative distribution of the probe, as mean ±s.e.m. for N =5 observations. See Methods for definition of NAWI. Inset is magnified for the thigh muscle tissues, showing a ~6.9 × increase in the probe accumulation at the site of infection. ( e – j ) Microscopy analysis of excised muscle tissue. ( e – g ) Bright-field images, with Gram staining. ( h – j ) Fluorescence images, using a green dye labelled on the M13. ( e , h ) The left muscle (control PBS injection) shows no evidence of Gram-positive S. aureus bacteria and negligible green fluorescence. ( f , i ) The right muscle (site of infection) shows the presence of clumps of violet-stained cocci of S. aureus . There is marked enhancement in the fluorescence intensity in the regions of large bacterial infection. Insets to parts of f and i , indicated by the red boxes, are shown in g and j respectively, at × 100 magnification. In g , individual cocci, ~0.5–0.8 μm in diameter are resolved. In j , the more heavily infected area shows brighter fluorescence compared with the less infected region. See Supplementary Fig. 7 and Supplementary Note 7 of Supplementary Information for additional analysis. Scale bar, 67.5 μm ( e , f , h , i ) and 13.7 μm ( g , j ). Full size image Moreover, to investigate the distribution of the probe injected into the circulation, we excised organs from the mice and imaged them for fluorescence signal ( Fig. 3c ). Shown are sample RoI maps of the spleen (Sp), stomach (St), liver (Li), kidneys (Ki), intestine (It), bladder (Bl), heart (Ht) and lungs (Lu). For comparison, we define a metric called the normalized area-weighted intensity (NAWI), a dimensionless quantity. We note here that other groups of researchers have defined their own metrics for calculating the biodistribution of injected fluorescent molecular probes. For example, Ning et al . [16] have used ‘Fluorescence Units per gram’ as a metric, obtained by measurements of the fluorescence signal of the excised organs homogenized in RIPA buffer. Liu et al . [17] , [31] have used ‘% Injected Dose per gram’, by collecting blood and tissue lysate samples at various time points p.i. These methods would be difficult to adopt exactly in our present study, due to the nature of the M13-SWNT probe and the possibility of SWNTs getting unconjugated from the M13 complex on using harsh mechanical treatments such as homogenization, ultrasonication and buffer dissolution techniques employed by the aforementioned groups. Therefore, we propose the NAWI (see Supplementary Fig. 5 and Supplementary Note 5 for the detailed procedure, and Methods for calculation) as a semi-quantitative metric that is designed to give an estimate of the relative distribution of the SWNT probe in various organs, rather than accurate absolute values of probe uptake. The NAWI is plotted in Fig. 3d , with the inset showing a part of the chart magnified for the right thigh and left thigh muscle tissues. We observe several interesting trends in Fig. 3d . First, there is a ~6.9 × increase in probe localization in the right thigh muscle at the site of infection, compared with the left thigh PBS control injection. This compares with the ~3.4 × enhancement calculated in the RoI analysis of the whole-animal images, shown in Fig. 2f . The higher value obtained in the excised tissue may be attributed to the significantly less scattering and background tissue autofluorescence [20] , [21] interfering with the SWNT signal in ex vivo analysis. Second, for the other organs, the maximum uptake is observed in the liver and spleen, ~50.2 × and ~2.4 × , respectively, compared with that of the left thigh tissue. This is an expected result, with several groups reporting similar observations [31] , [32] , and correlates to the large mass of the liver compared with the other organs. Finally, we see non-negligible probe distribution in the stomach, kidneys and intestine. This may be rationalized by the proposed mechanism of clearance [31] of functionalized SWNTs from the circulation by the mononuclear phagocyte system, mainly via the biliary pathway in faeces, with some excretion of SWNTs in urine at early time points p.i. We also evaluated the fluorescence stability of the SWNT probe, as a function of time, in vivo and in excised tissue. Supplementary Fig. 6 and Supplementary Note 6 discuss the findings. Over the 96-h duration of the experiment, the SWNT probe is distinguishable with a fluorescence signal ~85% of the peak intensity ( Supplementary Fig. 6a–d and Supplementary Note 6 ). Ex vivo , the tissues and organs retain up to >91% of their peak intensity at t =5 days post excision. We therefore expect minimal change in signal intensity for the purposes of calculating the NAWI, as the procedure is performed at t =1 day post excision. To confirm targeting, tissue samples from the thigh muscles were Gram stained, to detect Gram-positive S. aureus bacteria. Representative bright-field colour images are shown in Fig. 3e–g . In the left thigh ( Fig. 3e ), we see no evidence of staining. In contrast, Fig. 3f , a section of the right thigh, shows the presence of large clumps of crystal violet-stained S. aureus . Inset (red box, Fig. 3g ) shows a × 100 magnification, in which individual cocci, ~0.5–0.8 μm in diameter, are resolved, similar to reported images of S. aureus infections [33] . We infer that the bacterial infection is localized at the site of injection and, therefore, the NIR-II fluorescence signal enhancement may be attributed to a targeting of the bacteria by the SWNT-based probe. To further verify the co-localization of the anti- S . aureus -M13-SWNT probe at the site of infection, we additionally labelled the M13 virus with a green dye. Figure 3h–j show fluorescence images of the same sections as Fig. 3e–g . We observe negligible nonspecific signal in the left thigh tissue ( Fig. 3h ). In comparison, we see a significant increase in the fluorescence intensity at the region of heavy bacterial infection in Fig. 3i . Inset (red box, Fig. 3j ) at × 100 magnification evidently fluoresces much brighter. To compare the extent of colocalization, we performed Pearson’s correlation analyses comparing the bright-field Gram-stained images with the green fluorescence signal ( Supplementary Fig. 7 and Supplementary Note 7 ). We obtain a high Pearson’s correlation coefficient of 0.704±0.053, leading us to conclude that the anti- S.aureus -M13-SWNT probe is specifically targeting and localizing at the site of the bacterial infection. Comparison of SWNT probes with dye fluorophores Several groups have proposed that SWNT-based NIR-II imaging, compared with other NIR-I fluorophores such as dyes or quantum dots, is capable of achieving superior resolution at greater depths in tissue [17] , [18] , [20] , [24] , [26] . However, there has been very limited application of SWNTs for in vivo imaging, and there has been no reported study of using SWNTs as bacterial probes till date. In contrast, numerous studies [13] , [14] , [15] , [16] have used fluorescent dyes for targeting and imaging bacterial infections. We therefore compared the performance of our M13-SWNT probe versus dye-based fluorescence imaging techniques ( Fig. 4 ). For this, we performed experiments using two models of phantoms: (1) a hard polymer phantom, which was custom-designed to mimic the optical properties of human breast tissue and (2) a soft phantom, chicken tissue (see Methods). As a model NIR-I dye, we used Alexa Fluor 750, commonly used in in vivo imaging studies. We placed a capillary tube with a fluorophore (M13-Dye or M13-SWNT) at suitable depths inside the phantom and fluorescence images were taken by normal excitation on the top surface. 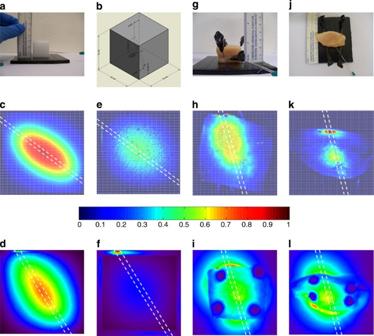Figure 4: Comparison of SWNT NIR-II imaging with NIR-I dye imaging using Alexa Fluor 750. Two models were studied: a hard optical phantom (a–f) and soft chicken tissue (g–l). The optical phantom used was a 3-cm cube, with a through-hole designed to fit a 1.65-mm diameter capillary tube, shown in the (a) photograph and the (b) CAD render. The capillary tube was filled with a fluorescent probe (M13-Dye or M13-SWNT) and placed parallel to the top face at a depth of 1 cm (c,d) or 2 cm (e,f). Chicken tissue was cut into cuboid shape and was used to place the fluorophore-containing capillary at a depth of (g) 1 cm and (j) 2 cm below the top surface. Samples were excited at normal incidence on the top face. (c,e,h,k) The SWNT images. (d,f,i,l) The corresponding dye images for the same geometries. The position of the capillary tube is indicated using the white dashed lines. All images were taken at detector saturation and normalized to the same 0–1 intensity scale. The lower signal spread and higher amplification ratio achieved using the SWNT probe (Table 1) indicates that it is better suited for high-resolution optical imaging at greater depths in tissue, compared to conventional dye fluorophores. Figure 4: Comparison of SWNT NIR-II imaging with NIR-I dye imaging using Alexa Fluor 750. Two models were studied: a hard optical phantom ( a – f ) and soft chicken tissue ( g – l ). The optical phantom used was a 3-cm cube, with a through-hole designed to fit a 1.65-mm diameter capillary tube, shown in the ( a ) photograph and the ( b ) CAD render. The capillary tube was filled with a fluorescent probe (M13-Dye or M13-SWNT) and placed parallel to the top face at a depth of 1 cm ( c , d ) or 2 cm ( e , f ). Chicken tissue was cut into cuboid shape and was used to place the fluorophore-containing capillary at a depth of ( g ) 1 cm and ( j ) 2 cm below the top surface. Samples were excited at normal incidence on the top face. ( c , e , h , k ) The SWNT images. ( d , f , i , l ) The corresponding dye images for the same geometries. The position of the capillary tube is indicated using the white dashed lines. All images were taken at detector saturation and normalized to the same 0–1 intensity scale. The lower signal spread and higher amplification ratio achieved using the SWNT probe ( Table 1 ) indicates that it is better suited for high-resolution optical imaging at greater depths in tissue, compared to conventional dye fluorophores. Full size image Figure 4a,b show respectively the photograph and an isometric view of the three dimensional computer aided design (3D CAD) render of the hard optical phantom. The precision machined hard phantom allows us to place the fluorophore-containing capillary at a depth of either 1 cm ( Fig. 4c,d ) or 2 cm ( Fig. 4e,f ) below the top surface. Figure 4g,j show the photographs of two pieces of chicken breast tissue, used as soft phantoms. In Fig. 4h,i , the fluorophore was inserted at a depth of 1 cm, while for Fig. 4k,l it was located at a depth of 2 cm. To compare the images of dye and SWNT fluorescence, we performed RoI analyses. All images were taken at detector saturation. After normalizing the images to the same 0–1 intensity colour scale (0 being dark, 1 being saturation), a threshold cutoff intensity was set at 0.35 for defining the RoI in each image. This cutoff was chosen to be sufficiently high such that the RoIs for all samples were encompassed within the specimen under consideration. To simplify the discussion, we pairwise compare the SWNT images with the corresponding dye images at the same depth ( Fig. 4c–d, e–f, h–i and k–l ,), for both types of phantoms. From the RoI images, we used two semi-quantitative metrics for evaluating the fluorophore characteristics, listed in Table 1 . First, we computed the RoI area as a measure of the ‘signal spread’. We observe that for the hard cube phantom, at 1 cm depth, the dye and SWNT have nearly equal signal spread. At 2 cm depth, however, the dye maintains an almost similar signal spread, while the SWNT signal gets sharper with an area of ~0.49 × of the dye spread. This contrast becomes more evident in the soft chicken tissue, where the SWNT signal is confined to an area of ~0.38 × and ~0.08 × that of the dye spread, for the 1 and 2 cm cases, respectively. Second, we calculated the ratio of the peak intensity of the signal to the average intensity over the RoI, or the ‘amplification ratio’. The amplification ratio is similar for the dye and SWNT in the hard phantom, ~1.6 and ~1.3 for the 1 and 2 cm cases, respectively. However, for the chicken, which is more representative of realistic tissue, with inhomogeneities such as fat, water and blood vessels, we observe a much higher amplification in the SWNT signal, ~1.4 × that of dye. Visually, without additional image processing, we are able to discern the finer aspects of the underlying sub-surface morphology of tissue in the SWNT-based images of the chicken, while such details are lost in the dye images. This may be attributed to the reduced tissue autofluorescence background in the NIR-II domain, and also to the less scattering due to haemoglobin and water molecules [21] . These phantom models show encouraging results towards achieving sharper feature resolution with lower background noise, and can form the foundation for further exploration of targeting and detection of localized, deeply buried infectious diseases in the body, using SWNT probes. In addition, we show that the SWNT probe is capable of binding to a biofilm model using a plate assay ( Supplementary Fig. 8 and Supplementary Note 8 ). However, more work is needed in this direction to ascertain the penetration capability and diffusion kinetics of the probe material in the biofilm matrix, which acts as a barrier defense mechanism. This can form the basis for future investigation towards the application of these SWNT probes for bacterial biofilm infections. Table 1 Signal spread (areal) and amplification ratio (peak/average intensity) for phantoms. Full size table Deep-Tissue in vivo imaging of bacterial endocarditis Infective endocarditis is a rapidly progressing, destructive infection of the heart valves, caused by bacteria that enter the bloodstream and settle in the heart lining, a heart valve or a blood vessel. This disease is associated with high mortality rates of ~15–47% (refs 34 , 35 ), with S. aureus being the most common infective pathogen [34] , and therefore there is a clinical need to be able to reliably diagnose S. aureus endocarditis infections. In this work, we used an established mouse model of S. aureus endocarditis [36] that consists of aortic valve bacterial vegetations, similar to those in humans. Under anaesthesia, the right carotid artery was isolated and a ~1.2–1.4 cm segment of suture was embedded down the artery into the heart, to cause damage to the aortic valve. This model resembles the presence of foreign material such as catheters, one of the major causes of infections in humans. The time of insertion of the suture was taken to be t =0. At t =24 h post insertion of the suture, the animals received the S. aureus Xen-29 strain through a tail vein injection. At t =48 h, the animals were imaged using the IVIS instrument to detect bioluminescence of the S. aureus infection (see Methods for details). 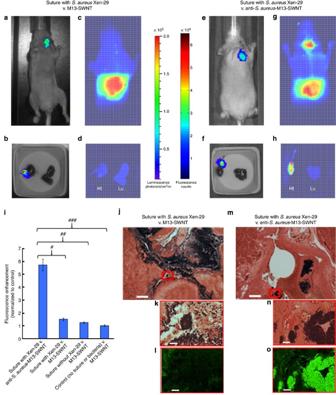Figure 5: Detection of deep-tissue infective endocarditis using the SWNT probe. Comparison of thein-situbioluminescence (a,b,e,f) from theS. aureusstrain Xen-29, with the NIR-II fluorescence from the SWNT probe (c,d,g,h). Also shown are the excised heart and lungs, obtained after euthanizing the animals;Ht: Heart,Lu: Lungs. (a–d) One representative animal is shown from the cohort that received the non-targeted M13-SWNT probe, while (e–h) illustrates an animal from the group that received the targeted anti-S. aureus-M13-SWNT probe, showing high specificity of detection. (i) Intensity enhancement of the fluorescence signal over the RoI, normalized to the control case (naive mice, without suture or bacterial injection, with M13-SWNT dosing). Data plotted as mean±s.d. forN=5 measurements for every set. #, ##,###P<0.01; statistically significant using Student’st-test. (j–o) Microscopy analysis of the excised heart tissues, showing bright-field images with Gram staining (j,m,k,n) and fluorescence images using a green dye labelled on the M13 (l,o). Gram staining shows the formation of large vegetations of Gram-positiveS. aureusinjandm. Parts of these images, indicated by the red boxes, are shown at × 100 magnification. There is marked enhancement in the fluorescence at the site of bacterial infection for the targeted anti-S. aureus-M13-SWNT-Alexa Fluor 488 case. Scale bar, 100 μm (j,m) and 20 μm (k,l,n,o). Figure 5a,e show representative images of the infection in the thoracic region. Only animals with detectable levels of infection were continued in the study, by dosing them with the SWNT-based probe through a retro-orbital injection. Next, at t =72 h p.i., the animals were imaged using our custom-built NIR-II fluorescence imaging instrument. Figure 5: Detection of deep-tissue infective endocarditis using the SWNT probe. Comparison of the in-situ bioluminescence ( a , b , e , f ) from the S. aureus strain Xen-29, with the NIR-II fluorescence from the SWNT probe ( c , d , g , h ). Also shown are the excised heart and lungs, obtained after euthanizing the animals; Ht : Heart, Lu : Lungs. ( a – d ) One representative animal is shown from the cohort that received the non-targeted M13-SWNT probe, while ( e – h ) illustrates an animal from the group that received the targeted anti- S. aureus -M13-SWNT probe, showing high specificity of detection. ( i ) Intensity enhancement of the fluorescence signal over the RoI, normalized to the control case (naive mice, without suture or bacterial injection, with M13-SWNT dosing). Data plotted as mean±s.d. for N =5 measurements for every set. #, ##, ###P <0.01; statistically significant using Student’s t -test. ( j – o ) Microscopy analysis of the excised heart tissues, showing bright-field images with Gram staining ( j , m , k , n ) and fluorescence images using a green dye labelled on the M13 ( l , o ). Gram staining shows the formation of large vegetations of Gram-positive S. aureus in j and m . Parts of these images, indicated by the red boxes, are shown at × 100 magnification. There is marked enhancement in the fluorescence at the site of bacterial infection for the targeted anti- S. aureus -M13-SWNT-Alexa Fluor 488 case. Scale bar, 100 μm ( j , m ) and 20 μm ( k , l , n , o ). Full size image We evaluated the ability of our SWNT-based probe to detect, and image with high specificity, the presence of infection in the heart valves, as shown in Fig. 5 . The left group of images in Fig. 5a–d shows a representative subject from the cohort, which received the non-targeted M13-SWNT probe. Although the presence of S. aureus infection is clearly detected through the bioluminescence from the bacterial strain, the NIR-II fluorescence signal is negligible in the thorax, other than that in the abdominal area. In contrast, the right group of images in Fig. 5e–h depicts a subject in the group that received the targeted anti- S. aureus -M13-SWNT probe, which illustrates a strong presence of NIR-II fluorescence signal at the surgical site. To further verify that the NIR-II fluorescence signal originates from the site of suture insertion in the heart, animals were euthanized and the organs were collected for imaging. Figure 5b,d,f,h show that although the bacterial infection is indeed present in both groups, only the targeted case shows strong fluorescence signal. The complete set of organs (heart, lungs, liver, spleen, kidneys, bladder, intestine, stomach and thigh muscle) was harvested and imaged for presence of bacterial infection ( Supplementary Fig. 9 and Supplementary Note 9 ), as well as to study the relative distribution of the SWNT probe in the body ( Supplementary Fig. 10 ). There is very little fluorescence signal from the lungs ( Supplementary Note 10 ), suggesting the probe localization to be at the site of suture insertion, leading to the bacterial infection in the heart. The above results are summarized in Fig. 5i , which plots the relative intensity enhancement of the NIR-II fluorescence signal. In addition to the above cases, we also performed two sets of control experiments. In one group, animals were embedded with the suture but were not induced with bacterial infection, followed by dosing with the SWNT probe. In a second control group, naive mice (without suture placement and without bacterial injection) were dosed with the SWNT probe. We observe that the targeted probe offers highly specific detection of this deep-tissue endocarditis infection model (Suture with Xen-29 v. anti- S. aureus -M13-SWNT) with a ~5.7 × enhancement in the fluorescence intensity over the control, which corresponds to a ~3.8 × increase compared with the nonspecific case (Suture with Xen-29 v. M13-SWNT). We also studied the colocalization of the SWNT probe at the site of the bacterial endocarditis, using green fluorescent dye labelled on the M13 virus. Figure 5 shows representative bright-field and fluorescent images taken on the same section, with the left group of images, Fig. 5j–l , from a subject receiving the non-targeted M13-SWNT-Alexa Fluor 488 probe and the right group Fig. 5m–o receiving the targeted anti- S. aureus -M13-SWNT-Alexa Fluor 488. In both cases, the formation of large clumps of bacterial vegetations is evident, in the low magnification images Fig. 5j,m , similar to that reported in literature [34] , [36] . At × 100 magnification, we see individual clumps of violet-stained cocci of S. aureus. The presence of large fluorescence colocalization in Fig. 5o at the site of bacterial infection provides additional evidence of the targeting of the SWNT probe, although we observe negligible fluorescence in the nonspecific M13-SWNT case in Fig. 5l . These findings provide further evidence of the applicability of the SWNT probes for in vivo targeting and detection of localized, deeply buried infectious diseases in the body. In summary, we present an application of carbon nanotube probes, for in vivo targeting and fluorescence optical imaging of bacterial infections. Using genetically engineered M13 virus as a multifunctional vector, we synthesize NIR-II fluorescent SWNT probes (M13-SWNT), with additional functionalization on the virus for active targeting of bacterial infections. We show highly specific targeting of S. aureus infections in live subjects, using these SWNT probes. Our SWNT probes offer distinct advantages of being biologically functionalized without surface chemical modification of SWNTs, for retaining high photoluminescence; aqueous dispersed, for in vivo applicability; actively targeted, for highly specific detection; modularly tunable, for detection of a wide range of pathogens; and low dosage achieving high contrast detection, for minimizing patient exposure. In addition, using breast tissue phantoms and chicken tissue, we demonstrate that these SWNT probes have the potential to offer better feature fidelity at greater depths, as quantified by the lower areal spread and higher amplification ratio compared with conventional NIR-I dye fluorophores. Finally, based on an endocarditis model of infection, we illustrate an example of deep-tissue in vivo imaging using the SWNT probes. These results open up exciting new opportunities for the development of NIR-II imaging using SWNT probes as a safer, non-ionizing, relatively less expensive alternative imaging modality, for non-invasive detection and monitoring of infectious diseases in the body. Preparation of the SWNT probe As-synthesized, non-functionalized HiPCO SWNTs (NanoIntegris, CA, USA) were dispersed in 2%(w/v) aqueous sodium cholate (SC-SWNTs), ultrasonicated for 10 min and centrifuged at 30,000 r.p.m. for 4 h to get well-dispersed SWNTs. The SWNT concentration of the supernatant was calculated using Beer-Lambert’s Law, where the extinction coefficient of HiPCO SWNT at 632 nm, ε 632 nm =0.036 l mg −1 cm −1 (or absorbance, A 632@1 cm × 27.8=[SWNTs] in μg ml −1 ). We used M13 virus to bind and stabilize SWNTs using a method reported previously [27] . M13 virus was amplified to a concentration of 3 × 10 13 pfu ml −1 (plaque forming units per ml). For the complexation, SC-SWNTs were mixed with phage in 1:1 ratio, to form M13-SWNT. Cell lines and culture The ability of M13-SWNT to selectively bind to different strains of bacteria was studied. We used strains of E. coli and S. aureus for this purpose. E. coli of two different strains, DH5-α (New England Biolabs, MA, USA) and JM109 (Promega, WI, USA) were used, of which the former lacks F′ -pili, the latter is F′ -positive. We also used Xen-29 strain of S. aureus (Caliper Life Sciences, MA, USA). All bacteria were grown in LB broth, with 50 μg ml −1 tetracycline for the E. coli strains and 50 μg ml −1 kanamycin for the S. aureus . The bacteria were grown in an incubator at 37 °C under vigorous shaking at 250 r.p.m. Steady-state log-phase growth was attained within 3–4 h of subculture, and growth was stopped when optical density 600 absorbance measurement attained a value of 0.5. One-step tunability of the SWNT probe To enable the SWNT probe to selectively target F′ -negative strains of bacteria, we used a modular one-step tuning process. Previously [19] , a method has been reported to express biotin acceptor peptide (BAP), GLNDIFEAQKIEWHE [37] , on the p3 coat protein of M13. M13 viruses expressing BAP (BAP-M13) were then enzymatically biotinylated at the lysine residue (Lys10) using a biotin-protein ligase (Avidity, CO, USA). The biotinylated peptide acts as a handle and allows for site-specific conjugation of streptavidin-modified targeting moieties. In the present application, antibodies against bacteria were attached to the BAP-M13 complex, and used to develop anti-bacterial antibody-M13-SWNT probes for targeting specific bacterial infections. Whole-animal imaging using the SWNT probe All animal handling and procedures were done in compliance with the Institutional Animal Care and Use Committee protocols. Procedures were pre-approved by MIT’s Committee on Animal Care. Female nude nu/nu mice, 43–56 days old were used (Charles River Laboratories, MA, USA). Two sets of experiments were performed, involving E. coli and S. aureus strains. For each strain, 2 groups of N =5 mice were studied. In the first set, one group received the DH5-α strain and the second group received JM109. In the second set, all mice received the Xen-29 strain. Cells (10 8 ) of bacteria in 50 μl LB media were injected in the right caudal thigh muscle using a 25-gauge needle. As negative control, 50 μl of 1 × PBS was also injected in the left thigh of each subject. After incubating, the bacteria in the living host for 1 h, 200 μl of the appropriate SWNT probe (or equivalently, a dosage of 0.232 mg kg −1 , for an average body weight ~25 g for mice) was injected into the circulation through a retro-orbital injection. The time of injection of the probe was taken as t =0. Post injection, mice were imaged at t =8 h or 24 h using a custom-built NIR-II fluorescence imaging instrument reported previously [19] (see Supplementary Fig. 3a and Supplementary Note 3 ). After this imaging sequence, mice were euthanized by CO 2 inhalation. For ex vivo analysis, we collected muscle tissue from the right flank (site of bacterial infection) and left flank (control PBS injection). These tissues (as excised) were imaged on the NIR instrument. Other organs recovered and imaged were the spleen, liver, kidneys, bladder, stomach, intestine, heart and lungs. After imaging, the parts were fixed in 10% formalin and mounted in paraffin wax. For comparing the relative distribution of the probe in the various organs, we define a dimensionless metric, the NAWI, calculated as follows. The procedure for preparing the tissue slices for calculating the NAWI is described in detail in Supplementary Note 5 . From the NIR-II fluorescence images such as in Supplementary Fig. 5 , we integrated the total fluorescence intensity I ij , total for each slice, as where I ijk ( x k , y k ) is the signal intensity corresponding to a pixel ( x k , y k ) in the 320 × 256 detector array for the j th slice in the i th tray, and only pixels with a readout higher than a certain threshold intensity I th are considered. Larger organs, such as the liver, require more sections, such as 12 trays in Supplementary Fig. 5b , while smaller tissues such as thigh muscle require only 2 trays, as in Supplementary Fig. 5e . We used a cutoff threshold of 35% of peak intensity for each organ. As our NIR-II imaging technique is a two-dimensional planar projection, we used an Areal density ρ ij , Areal , (instead of volumetric density), defined as mass/area, where m ij is the mass of the the j th slice in the i th tray, and the area of the slice is the sum of the total number of pixels in the RoI, that is, for which I ijk ( x k , y k )≥ I th . Using the areal density, we get an estimate of the mass of the SWNT probe present in each organ, as Finally, we normalize all values with respect to M probe of the left thigh (control PBS injections), to get a dimensionless number, the Microscopy analysis Five-micrometre-thick tissue sections were mounted on glass slides and stained with Gram staining kit (Sigma-Aldrich, St Louis, MO). They were observed with a Zeiss Axioplan II upright microscope with objective lenses of × 20 (air) and × 100 (oil immersion) magnification. Further, to determine the localization of the targeted SWNT probe at the site of bacterial infection, we used M13 labelled with a green fluorescent dye, Alexa Fluor 488 (Life Technologies, NY, USA). The anti- S. aureus -M13-SWNT-AlexaFluor488 probe was injected into the infected mice, and after imaging and killing the animals tissue sections were obtained. The samples were treated for 24 h with ProLong Gold antifade reagent (Invitrogen Molecular Probes, OR, USA), followed by Gram staining. Fluorescence images were taken using a EXFO-X-cite fluorescence illumination source and a Cy2 fluorescence filter cube paired with a Hamamatsu Orca ER1394 monochrome camera, with colocalized bright-field images. Phantom measurements To evaluate the imaging characteristics of the SWNT probe compared with commercially available fluorescent dyes, we used two models—a hard phantom and soft tissue. We tested both models using Alexa Fluor 750 (Life Technologies), a common NIR-I dye with a peak emission at λ =789 nm, conjugated to the M13 virus (M13-Dye), and with our NIR-II M13-SWNT probe. M13-Dye images were taken on an IVIS Spectrum instrument (Caliper Life Sciences, MA, USA), while M13-SWNT images were obtained using our custom NIR-II imager. First, we used a polymer phantom designed to mimic the optical characteristics of human tissue (Biomimic, INO, Quebec, Canada). This phantom has an absorption coefficient μ a =0.1 cm −1 and a scattering coefficient μ s =14 cm −1 at λ =690 nm. The hard phantom was custom fabricated as a 3 cm × 3 cm × 3 cm cube, with a 1.65-mm diameter cylindrical through-hole running parallel to one face, at a depth of 1 cm below the said face (see Fig. 4b ). Capillary tubes, with an outer diameter of 1.65 mm, were used to load fluorophore (M13-Dye or M13-SWNT). Second, to have a more realistic model of tissue, we used chicken breast meat available off the shelf in grocery stores (Star Markets, MA, USA). We repeated the same measurements using capillary tubes, with two pieces of breast meat, cut into approximate cuboids. In one instance, the fluorophore was inserted at a depth of 1 cm ( Fig. 4g–i ) and in the second case, it was located at a depth of 2 cm ( Fig. 4j–l ). Deep-tissue in vivo imaging of bacterial endocarditis Mice were anaesthetized under flowing isoflurane. A surgical microscope (Nikon SMZ-1000, Japan) paired with a NI-150 150W high-intensity illuminator (Nikon Instruments, Inc., Japan) coupled through a beamsplitter to a SPOT Idea 5Mp Color Mosaic color camera (Diagnostic Instruments Inc., WI, USA) was used. The right carotid artery was gently separated from the neurovascular bundle and isolated with two strands of 6–0 silk, and a ~1.2–1.4 cm segment of suture material (4–0, Ethicon) was inserted through a small incision in the carotid artery down to the level of the aortic valve and left in place. The time of the suture insertion surgery was taken as t =0. The analgesic used was buprenorphine, at a dose of 0.05–0.1 mg kg −1 administered pre-surgery and also at regular intervals of 6–12 h, for 3 days post surgery. In addition, warm sterile 0.9% saline was given subcutaneously at a dose of 20 ml kg −1 of body weight, for hydration. Mice were allowed to recover for 24 h Next, at t =24 h, 5 × 10 6 cells of the Xen-29 strain of S. aureus in 50 μl LB medium were injected through the tail vein, using a 26-gauge needle. The bacteria were incubated for 24 h to induce the endocarditis infection, which was then monitored through bioluminescence imaging of the Xen-29 strain ( Fig. 5a,e ) using the IVIS instrument. Only animals with detectable levels of infection in the thoracic region were continued through the experiment; the rest were humanely euthanized. At t =48 h, 200 μl of the appropriate SWNT probe (or equivalently, a dosage of 0.232 mg kg −1 , for an average body weight ~25 g for mice) was injected into the circulation through a retro-orbital injection. Finally, at t =72 h, the subjects were imaged using the NIR-II fluorescence imaging instrument. After this imaging sequence, animals were euthanized by CO 2 inhalation. We collected the organs, including the heart, lungs, liver, spleen, kidneys, bladder, intestine, stomach and thigh muscle tissue (see Supplementary Fig. 9 ). These were used to evaluate the systemic spread of the bacteria following the tail vein injection and to validate that the infection is localized in the heart. In addition, the excised organs were used to determine the relative distribution of the probe, using the NAWI method described above ( Supplementary Fig. 10 ). Five-micrometre-thick transverse sections of the heart tissue, normal to the point of insertion of the suture in the carotid artery, were taken at step intervals of 50 μm to study the presence of bacterial vegetations. Gram-stained sections were observed under light and fluorescence microscopes to provide further evidence of targeting of the SWNT probe. For the purpose of this study, four sets of animals were used ( N =5 each). Two of the groups received the suture with the bacteria, with one of them receiving the targeted probe (anti- S. aureus -M13-SWNT) and the other receiving the non-targeted case (M13-SWNT). In addition, two other control groups ( N =5 each) were studied, with one group receiving the suture, but no bacteria, with M13-SWNT dosing, and the last group consisting of naive mice (no suture or bacteria) with M13-SWNT dosing. To further verify the co-localization of the SWNT probe at the site of endocarditis infection, we injected probes labelled with an additional green fluorescent dye, Alexa Fluor 488. After imaging and euthanizing the animals, the tissues were harvested and fixed in formalin. Five-micrometre-thick transverse sections were taken from the heart muscle tissue, normal to the point of insertion of the suture. The sections were stained with crystal violet to identify Gram-positive bacteria and counterstained with safranin. How to cite this article: Bardhan, N. M. et al . Carbon nanotubes as in vivo bacterial probes. Nat. Commun. 5:4918 doi: 10.1038/ncomms5918 (2014).